A versatile source of single photons for quantum information processing The generation of high-quality single-photon states with controllable narrow spectral bandwidths and central frequencies is key to facilitate efficient coupling of any atomic system to non-classical light fields. Such an interaction is essential in numerous experiments for fundamental science and applications in quantum communication and information processing, as well as in quantum metrology. Here we implement a fully tunable, narrow-band and efficient single-photon source based on a whispering gallery mode resonator. Our disk-shaped, monolithic and intrinsically stable resonator is made of lithium niobate and supports a cavity-assisted spontaneous parametric down-conversion process. The generated photon pairs are emitted into two highly tunable resonator modes. We verify wavelength tuning over 100 nm of both modes with controllable bandwidth between 7.2 and 13 MHz. Heralding of single photons yields anti-bunching with g (2) (0)<0.2. The quantum state of a single-photon stands among the most fundamental and intriguing manifestations of quantum physics [1] . At the same time, single photons and pairs of single photons are important building blocks in the fields of linear optical based quantum computation [2] and quantum repeater infrastructure [3] . These fields possess enormous potential [4] , and much scientific and technological progress has been made in developing individual components, like quantum memories and photon sources using various physical implementations [5] , [6] , [7] , [8] , [9] , [10] , [11] . However, further progress suffers from the lack of compatibility between these different components. Ultimately, one aims for a versatile source of single photons and photon pairs to overcome this hurdle of incompatibility. Such a photon source should allow for tuning of the spectral properties (wide wavelength range and narrow bandwidth) to address different implementations while retaining high efficiency. In addition, it should be able to bridge different wavelength regimes to make implementations compatible. Here we introduce and experimentally demonstrate such a versatile single photon and photon pair source based on the physics of whispering gallery resonators. A disk-shaped, monolithic and intrinsically stable resonator is made of lithium niobate (LiNbO 3 ) and supports a cavity-assisted triply resonant spontaneous parametric down conversion (SPDC) process. Measurements show that photon pairs are efficiently generated in two highly tunable resonator modes. We verify wavelength tuning over 100 nm between both modes with a controllable bandwidth between 7.2 and 13 MHz. Heralding of single photons yields anti-bunching with g (2) (0)<0.2. This compact source provides unprecedented possibilities to couple to different physical quantum systems and renders it ideal for the implementation of quantum repeaters and optical quantum information processing. Basic concept It is known that in a nonlinear medium, a photon can spontaneously decay into a pair of photons, usually called signal and idler. This process, referred to as SPDC, preserves the energy and momentum of the parent photon. The resulting pair of photons possesses the ability to bridge different wavelength ranges. At the same time, detecting one photon of this pair unambiguously heralds the presence of a single photon. In principle, the process of SPDC has a very high bandwidth. By assisting it with a high-quality factor (high-Q) resonator, the desired narrow bandwidth of a few megahertz for the individual photons can be ensured [12] . A thorough description of this resonator-assisted SPDC leads to a two-mode EPR entangled state [13] and has successfully been used to generate heralded single photons [14] . Recently, resonator-assisted SPDC has led to a substantial progress towards an efficient narrow-band source [15] . However, the wavelength and bandwidth tunability remained a major challenge. We overcome this problem by using an optical whispering gallery mode resonator (WGMR). These resonators are based on total internal reflection of light and can be tuned to all wavelengths within the whole transparency range of the material they are made of [16] . WGMRs can have high-Q leading to narrow bandwidths [17] that match those of atomic transitions. Therefore, further spatial and spectral filtering [18] , [19] , [20] , which can drastically reduce the systems efficiency, becomes unnecessary. Recently, it was shown that the strong second-order nonlinearity in LiNbO 3 can be used in monolithic WGMRs for highly efficient nonlinear processes [21] , [22] , [23] , [24] , [25] . The heart of our experiment ( Fig. 1 ) is a crystalline WGMR with a high-quality factor on the order of Q ≈10 7 (ref. 22 ). The coupling of light to the resonator is realized via optical tunnelling between a diamond prism and the resonator. With a triply resonant configuration, we exploit natural phase-matching to achieve SPDC (see Methods). We verify the spontaneous regime of the parametric process by demonstrating a linear dependence of the pair production rate on the pump power ( Fig. 2 ). Correcting for the detection efficiency, we find a pair production rate of 1.3 × 10 7 pairs per second per mW pump power within a single spectral bandwidth of 13 MHz. This efficiency is two orders of magnitude higher than the one found in previous experiments [14] . 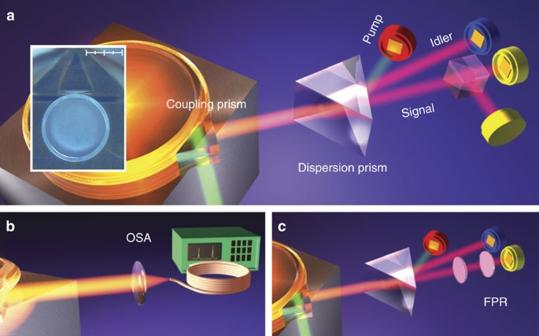Figure 1: Sketch of the experiment. (a) The WGMR manufactured from LiNbO3is pumped by a frequency doubled Nd:YAG laser emitting continuous wave light at a wavelength of 532 nm. A diamond prism allows for evanescent wave coupling to the resonator. In type-I PDC, correlated photon pairs can be created in resonator modes phase-matched with the pump. The intra-cavity pump power is chosen to be far below the OPO threshold determined in a previous experiment23. The signal and the idler photons (as well as the residual pump) are coupled out of the triply resonant WGMR using the same diamond prism and are separated by an additional dispersion prism. The idler photons are detected with one APD (blue). The signal photons are detected in a Hanbury Brown–Twiss setup, consisting of a 50:50 beamsplitter and two APDs (yellow). The residual pump is monitored with a PIN diode (red). Inset: A photomicrograph of the setup22. Scale bar, 2.0 mm. (b) To verify coarse tuning of the signal and idler wavelengths, the output of the WGMR is analysed with an OSA. (c) To verify fine-tuning of the wavelength, we use a scanning FPR in the signal arm. Figure 1: Sketch of the experiment. ( a ) The WGMR manufactured from LiNbO 3 is pumped by a frequency doubled Nd:YAG laser emitting continuous wave light at a wavelength of 532 nm. A diamond prism allows for evanescent wave coupling to the resonator. In type-I PDC, correlated photon pairs can be created in resonator modes phase-matched with the pump. The intra-cavity pump power is chosen to be far below the OPO threshold determined in a previous experiment [23] . The signal and the idler photons (as well as the residual pump) are coupled out of the triply resonant WGMR using the same diamond prism and are separated by an additional dispersion prism. The idler photons are detected with one APD (blue). The signal photons are detected in a Hanbury Brown–Twiss setup, consisting of a 50:50 beamsplitter and two APDs (yellow). The residual pump is monitored with a PIN diode (red). Inset: A photomicrograph of the setup [22] . Scale bar, 2.0 mm. ( b ) To verify coarse tuning of the signal and idler wavelengths, the output of the WGMR is analysed with an OSA. ( c ) To verify fine-tuning of the wavelength, we use a scanning FPR in the signal arm. 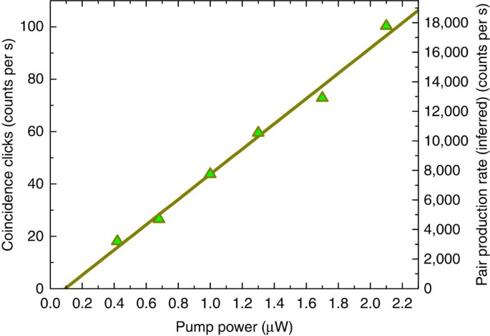Figure 2: Coincidences versus pump power. The coincidence clicks and the pair production rate depending on the pump power (each measurement time: 30 min; coincidence window: 30 ns). Full size image Figure 2: Coincidences versus pump power. The coincidence clicks and the pair production rate depending on the pump power (each measurement time: 30 min; coincidence window: 30 ns). Full size image Cross-correlations The quantum state of the emitted photons can be characterized by observing the temporal correlations of photon detection events between the signal and the idler arm, that is, the Glauber cross-correlation function (ref. 26 ) (see Supplementary Note 1 ). For a Lorentzian line shape, one can calculate that ( [12] , [27] ), where γ is the characteristic decay rate and R is the pair production rate. For an SPDC process enhanced by a high-Q resonator, such as our WGMR, the width of the correlation function is determined by the coherence time of the emitted photons corresponding to the bandwidth Δ ν = γ /2 π of the resonator. An exceptional feature of WGMRs is the widely and continuously tunable bandwidth Δ ν . This feature is accessible through the evanescent coupling, that is, by varying the distance between the coupling prism and the resonator. Note that for conventional resonators, this would require a tunable transparency of the resonator mirrors, which is very difficult to realize, especially for high-Q resonators. In addition, the change in the pump bandwidth will also modify the conversion efficiency. In Fig. 3a , we present the experimental data for . Using exponential fits (solid lines) to the data (dots), we find the correlation time and determine the bandwidth Δ ν , acquired for different coupling distances. We demonstrate a tunability of bandwidth between 7.2 and 13 MHz, which can in principle be extended drastically (see Supplementary Fig. S1 ). 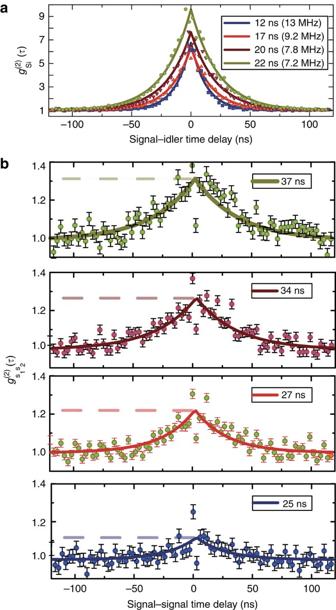Figure 3: Cross-correlation and autocorrelation. (a) Normalized cross-correlation functionsmeasured for different coupling distances of the WGMR. The bandwidth of the generated photons is determined by fitting an exponential (solid lines) to each measured data set (dots). The exponential fits demonstrate a bandwidth tunability of nearly a factor of 2, starting from the smallest experimentally verified bandwidth of 7.2 MHz. (b) Normalized autocorrelation functionmeasured for the same coupling distances as in the case of the cross-correlation function (keeping colour coding ofFig. 3a). Error bars are calculated assuming poissonian statistics of the individual measurement points. Figure 3: Cross-correlation and autocorrelation. ( a ) Normalized cross-correlation functions measured for different coupling distances of the WGMR. The bandwidth of the generated photons is determined by fitting an exponential (solid lines) to each measured data set (dots). The exponential fits demonstrate a bandwidth tunability of nearly a factor of 2, starting from the smallest experimentally verified bandwidth of 7.2 MHz. ( b ) Normalized autocorrelation function measured for the same coupling distances as in the case of the cross-correlation function (keeping colour coding of Fig. 3a ). Error bars are calculated assuming poissonian statistics of the individual measurement points. Full size image Autocorrelations In a next step, the number of effective modes in the generated states is estimated from the normalized Glauber autocorrelation function (see Supplementary Note 2 ). The value is expected to scale with the number of effective modes [28] , n as 1+1/ n . In Fig. 3b , autocorrelation functions are shown for the same coupling distances as the cross-correlation functions in Fig. 3a . The number of involved modes clearly depends on the distance between the prism and the resonator. By increasing this distance, the peak values increases up to a maximum of 1.35, which indicates three effective modes. We want to point out that this high quality is naturally achieved by our source without spectral and spatial filtering. In principle, efficient single-mode operation is feasible by optimizing the pump spectrum, and using even larger coupling distances or different resonator geometries, featuring a more sparse WGMR spectrum [17] . For the experimental data in Fig. 3b , the corresponding decay times are determined by fitting exponentials to each data set. We find that the decay times of the autocorrelation function exceed the decay times of the cross-correlation function by a factor between 1.7 and 2.0. A difference in decay times is already expected for a single-mode case [29] and was observed in previous resonator-assisted SPDC experiments [15] . Heralded autocorrelation To demonstrate heralded single photons, we evaluate the normalized Glauber autocorrelation function conditioned on an idler detection event (see Supplementary Note 3 ). The minimum of the function is sensitive to the non-classical signal-idler correlations and tends to zero for heralded single-photon states. In Fig. 4 , the special case of is presented with a heralding interval of 20 ns. The characteristic anti-bunching of is clearly visible, which reflects the non-classical correlations between two single photons in two different arms. 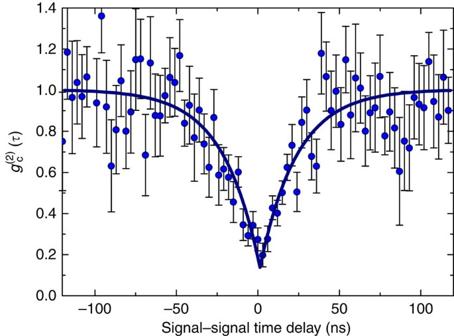Figure 4: Heralded autocorrelation. Normalized Glauber autocorrelation functionconditioned on an idler detection event with a heralding interval of 20 ns. The clearly visible anti-bunching dip proves the non-classicality of our heralded single-photon source. Error bars are calculated assuming poissonian statistics of the individual measurement points. Figure 4: Heralded autocorrelation. Normalized Glauber autocorrelation function conditioned on an idler detection event with a heralding interval of 20 ns. The clearly visible anti-bunching dip proves the non-classicality of our heralded single-photon source. Error bars are calculated assuming poissonian statistics of the individual measurement points. Full size image Wavelength tuning For compatibility with various components such as stationary qubits (for example, atomic transitions), non-classical light sources need to be tunable not only in bandwidth of the generated light but also in their central wavelength to match the qubit’s transition. In a triply resonant optical parametric oscillator (OPO), such wavelength tuning is realized by controlling the phase-matching. In our setup, we have control over the optical length of the resonator via the applied temperature and the voltage. Because of the limited sensitivity of the wavelength-measurement devices, the wavelength-tuning demonstration was carried out above the OPO threshold. 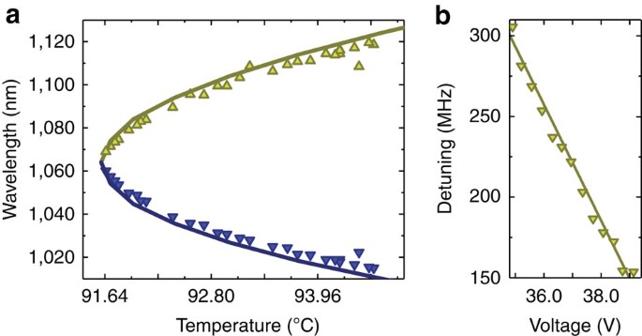Figure 5: Wavelength tuning. (a) By changing the resonator temperature over 3 °C, we measure a wavelength detuning of 100 nm between signal (yellow triangles) and idler (blue triangles) with an OSA. This agrees well with the phase-matching condition for WGMRs (solid line). (b) By changing the bias voltage over a range of 4 V, we measure a mode-hop free linear wavelength detuning of 150 MHz with a scanning Fabry–Perot interferometer (free spectral range of 1 GHz). Figure 5a shows the wavelength tuning measured with an optical spectrum analyzer (OSA) while the resonator temperature was changed (see Fig. 1b ). Varying the temperature over 3 °C results in a wavelength detuning of 100 nm between the signal and the idler. In Fig. 5b , we demonstrate a continuous fine-tuning of the central wavelength by applying a voltage across the WGMR. This measurement is realized by sending the signal beam to a scanning Fabry–Perot interferometer, as shown in Fig. 1c . By changing the bias voltage over a range of 4 V, we measure a mode-hop free wavelength detuning of 150 MHz, which potentially can be applied fast [30] . Figure 5: Wavelength tuning. ( a ) By changing the resonator temperature over 3 °C, we measure a wavelength detuning of 100 nm between signal (yellow triangles) and idler (blue triangles) with an OSA. This agrees well with the phase-matching condition for WGMRs (solid line). ( b ) By changing the bias voltage over a range of 4 V, we measure a mode-hop free linear wavelength detuning of 150 MHz with a scanning Fabry–Perot interferometer (free spectral range of 1 GHz). Full size image In conclusion, we have demonstrated a highly efficient SPDC process in a monolithic WGMR. With this configuration, we realized the narrow-band emission of heralded single photons whose bandwidth and wavelength can simultaneously be tuned. For the investigated crystalline resonator, we verify a bandwidth tunability between 7.2 and 13 MHz and a wavelength tunability of 100 nm between the down-converted fields. Operating our setup in a Sagnac configuration can transform it to a polarization entanglement source [31] . By changing the WGMR geometry and crystal doping and modifying the phase-matching temperature, one is readily able to address the wavelength of various atomic transitions and connect them to the telecom wavelengths (see Supplementary Note 4 ). If necessary, the modification of the WGMR geometry can be used to realize high bandwidth of the emitted photons (see Supplementary Note 5 ). This renders the source ideal for the implementation of quantum repeaters and quantum information processing in general. Experimental details Our WGMR is manufactured from a 5% MgO-doped LiNbO 3 wafer. The symmetry axis of the resonator coincides with the crystal’s optical axis. The system is similar to a triply resonant OPO but is operated far below its experimentally determined pump power threshold [23] . As a pump source, we use a continuous wave frequency doubled Nd:YAG laser (InnoLight, Prometheus) with a wavelength of 532 nm and a linewidth of 5 kHz. Typical pump powers at the input face of the coupling prism are on the order of several hundred nanowatts. The pump light is coupled to the resonator using a diamond prism and is coupled out together with the spontaneously generated signal and idler photons using the same prism. We match the pump laser to the WGMR by a sample and hold locking. During the 1-ms sample phase, we sweep the laser across the WGMR resonance and determine the resonance frequency by monitoring the pump transmission. During the 199-ms hold phase, the laser frequency is kept on the resonance. Natural type-I SPDC phase-matching is realized by stabilizing the resonator temperature at the appropriate set point. An additional fast control over the effective resonator length is realized by a voltage applied across the resonator. Planar electrodes are placed on the top and bottom side of the disk resonator. Although we did not explicitly lock the parametric modes in the WGMR, the parametric down-conversion process was sufficiently stable to enable measurements for more than 2 weeks. Finally, the signal and the idler are separated from each other and from the transmitted pump light using a dispersion prism and subsequently are directed to the detection stage. Measurement of the correlation functions To measure all three Glauber correlation functions, we use three avalanche photodiodes (APDs; id Quantique id400). The idler photons are detected with one APD, whereas the signal photons are detected in a Hanbury Brown–Twiss setup [32] (two APDs placed after a 50:50 beamsplitter). All APDs used in the experiment are operated in the Geiger mode and at a quantum efficiency of 7.5%. The electronic signals from the APDs are recorded by a time-to-digital converter (quTau; qutools GmbH), with a temporal resolution of τ d =162 ps. The time-to-digital converter records incoming detection events from the APDs with their time-stamps and channel number and streams the acquired data to a computer. From the raw time-stamps, the relative time delays were calculated using a software implemented start–stop algorithm. The bin size for all auto- and cross-correlation measurements was set to 3 ns. To avoid the influence of afterpulsing of the APDs on the statistics, we choose a slightly different dead time for each APD. The combination of low quantum efficiency and large deadtimes (≈10 μs) required to run the experiment for more than 2 weeks to present statistically significant results. Throughout the measurement period, the system is operated without active stabilization of the distance between the coupling prism and the WGMR. To have a measure of the coupling distance, we continuously recorded the pump-coupling efficiency, measured as the pump-transmission contrast during the sample phase. In the undercoupled regime, a decreasing contrast corresponds to an increased distance. By the virtue of the fact that the idler and the transmitted pump light exit the WGMR through the same coupling prism, we can sort the data according to the WGMR coupling distances, which determine the signal and idler bandwidths. Measurement of the wavelength tuning Besides the possibility of tuning the bandwidth of the generated single photons, our system has the ability to tune their central wavelengths. The effective resonator lengths for the involved modes are dependent on temperature and voltage, for example, due to thermo-refractive and electro-optical effects. This gives us control over the phase-matched wavelength triplet in the PDC process. The wavelength tuning based on the resonator bias voltage allows for a rapid and continuous (mode-hop free) tuning within over a hundred megahertz. Changing the resonator temperature allows for a slow tuning of each signal and idler over several tens of nanometres. To verify the wavelength tuning in the regimes mentioned, we use a scanning Fabry–Perot resonator (FPR) and an OSA. Because of the low sensitivity of these instrument’s sensors, we measured the signal and idler beams when operating above the OPO threshold. The tunability demonstration nonetheless remains valid because the phase-matching conditions do not depend on sub- or above threshold operation. Tuning based on variation of the resonator bias voltage We place a scanning FPR with a free spectral range of 1 GHz in the signal beam. While continuously modulating the bias voltage, we monitor the transmission through the FPR on an oscilloscope and find a tunability of the centre wavelength in the megahertz regime. The FPR is scanned over more than one free spectral range to calibrate the measurement results. Tuning based on variation of the temperature For the measurement of the wavelength tuning based on variation of the temperature, the dispersion prism is substituted by a polarization beamsplitter. Consequently, only the vertically polarized pump is separated from the horizontally polarized parametric beams. Signal and idler are jointly coupled to an optical multimode fibre and guided to the OSA, which allows us to confirm the tunability over several tens of nanomenters. For all temperatures, the pump laser is coupled to the same resonator mode, although with changing frequency. How to cite this article: Förtsch, M. et al . A versatile source of single photons for quantum information processing. Nat. Commun. 4:1818 doi: 10.1038/ncomms2838 (2013).